Electronic modulation of infrared radiation in graphene plasmonic resonators All matter at finite temperatures emits electromagnetic radiation due to the thermally induced motion of particles and quasiparticles. Dynamic control of this radiation could enable the design of novel infrared sources; however, the spectral characteristics of the radiated power are dictated by the electromagnetic energy density and emissivity, which are ordinarily fixed properties of the material and temperature. Here we experimentally demonstrate tunable electronic control of blackbody emission from graphene plasmonic resonators on a silicon nitride substrate. It is shown that the graphene resonators produce antenna-coupled blackbody radiation, which manifests as narrow spectral emission peaks in the mid-infrared. By continuously varying the nanoresonator carrier density, the frequency and intensity of these spectral features can be modulated via an electrostatic gate. This work opens the door for future devices that may control blackbody radiation at timescales beyond the limits of conventional thermo-optic modulation. Thermal radiation is commonly viewed to be broadband, incoherent and isotropic, with a spectral profile and intensity that are dependent on the emissivity of a material, and that vary only with changes in temperature. Recent experiments on nanoengineered structures, however, have begun to challenge these notions, showing that blackbody emission can be coherent and unidirectional, with narrow spectral features. These structures have included patterned gratings on metal or silicon carbide surfaces that can control the directionality and coherence of thermal radiation [1] , [2] , as well as photonic crystals [3] , size-tunable Mie resonances [4] and frequency-selective meta-surfaces [5] , which can tune the spectral profile. Progress has also been made in demonstrating dynamic control of thermal radiation through in situ modification of material emissivity. This has been achieved with devices that incorporate phase change materials, which display temperature-dependent emissivities [6] , as well as electronically controlled devices, where injected charges are used to overdampen polariton modes in quantum wells [7] . These results suggest that careful control of both the photonic and electronic structure of metasurfaces could allow for thermal emitters that have continuously variable frequency and directionality control, and that can operate at speeds much faster than typical thermal cycling times, potentially approaching speeds of modern telecommunication devices. Graphene provides a unique platform for studying and controlling thermal radiation at infrared wavelengths. The optical absorptivity/emissivity of graphene depends on two carrier density-dependent terms: an intraband contribution that is characterized by a large Drude-like peak in the DC to far-IR range, and an interband contribution that manifests as a step-like feature in the absorption in the far to near-IR [8] , [9] , [10] , [11] , [12] , [13] . In addition, the linear bandstructure and two-dimensional nature of graphene allow for it to support plasmonic modes that have a unique dispersion relation [14] , [15] , [16] , [17] . These plasmonic modes have been proposed as a means of efficiently coupling to THz radiation [18] , [19] , [20] , and they have been shown to create strong absorption pathways in the THz to mid-IR when the graphene is patterned to form plasmonic Fabry-Perot resonances [21] , [22] , [23] , [24] . The intensity and frequency of the plasmonic modes in graphene are carrier density dependent, and they display extermely large mode confinement, which allows them to efficiently couple to excitations (for example, phonons) in their environment and to create new optical modes [21] , [22] , [25] , [26] . As the graphene sheet is heated up, these different infrared absorption pathways become thermal emission sources, with contributions that vary with the graphene carrier density and surface geometry. The graphene plasmons are particularly interesting as thermal emitters because their small mode volumes allow for extremely efficient thermal energy transfer in the near field [27] , [28] , and also lead to large Purcell factors that can enhance the emission rate of emitters within the plasmon mode volume [29] . These large Purcell factors suggest that electronic control of the graphene plasmonic modes could potentially control thermal radiation at timescales much faster than the spontaneous emission rate for conventional light emitting diodes and classical blackbody emission sources. In the present work, we experimentally demonstrate the dynamic tuning of blackbody emission through electronic control of graphene plasmonic nanoresonators on a silicon nitride substrate at temperatures up to 250 °C. Our device is based on field effect tuning of the carrier density in nanoresonators, which act as antennas to effectively outcouple thermal energy within the resonator mode volume. We show that through this mechanism the thermal radiation generated by substrate phonons and inelastic electron scattering in graphene can be tuned on and off. By varying the charge carrier density of the graphene from 0 to 1.2 × 10 13 cm −2 , with resonator widths from 20 to 60 nm, we show that a narrow bandwidth emission feature may be tuned in intensity and varied in frequency across the mid-IR, from ∼ 1,200–1,600 cm −1 . Mid-IR graphene nanoresonator device geometry A schematic of the measurement apparatus and device geometry are shown in Fig. 1a (see Methods). The device consists of 20–60 nm wide graphene nanoresonators patterned into a graphene sheet on a 1 μm SiN x layer with a gold back reflector that also serves as a back gate electrode. This device geometry was previously used as a gate-tunable absorber in the mid-IR, where a large enhancement in absorption was observed when the graphene plasmonic resonance was matched to the energy of the λ /4 n SiN resonance condition in the 1 μm SiN x layer, which occurred at 1,360 cm −1 (refs 30 , 31 ) In those experiments, the polarized absorption in the graphene nanoresonators could be tuned from 0 to up to 24.5% for large carrier densities. In this work, a similar sample displayed up to 3% total absorption when probed using our apparatus. This smaller number reflects the use of non-polarized light, the higher numerical aperture objective of the apparatus, the effect of the window of the vacuum stage and the lower carrier densities used due to the onset of Poole-Frenkel tunnelling in the SiN x at higher temperatures and high gate biases (see Supplementary Note 1 ; Supplementary Figs 1, 2 and 3 for details) [30] , [32] . 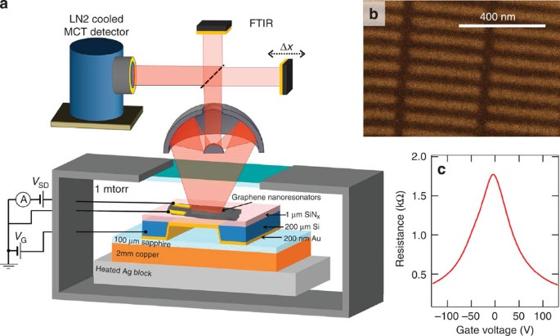Figure 1: Device and experimental set-up. (a) Schematic of experimental apparatus. The 70 × 70 μm2graphene nanoresonator arrays are placed on a 1 μm thick SiNxmembrane with 200 nm Au backreflector. The graphene was grounded through Au(100 nm)/Cr(3 nm) electrodes that also served as source-drain contacts. A gate bias was applied through the SiNxmembrane between the underlying Si frame and graphene sheet. The temperature-controlled stage contains a feedback controlled, heated silver block that held a 2 mm thick copper sample carrier, with a 100 μm thick sapphire layer used for electrical isolation. The temperature was monitored with a thermocouple in the block, and the stage was held at a vacuum of 1 mtorr. A 1 mm thick potassium bromide (KBr) window was used to pass thermal radiation out of the stage, which was collected with a Cassegrain objective and passed into an FTIR with an MCT detector. (b) A representative SEM image of 30 nm graphene nanoresonators on a 1 μm thick SiNxmembrane. (c) Source-drain resistance versus gate voltage curve of the device. The peak in the resistance occurs at the charge neutral point (CNP), when the Fermi level (EF) is aligned with the Dirac point. Figure 1: Device and experimental set-up. ( a ) Schematic of experimental apparatus. The 70 × 70 μm 2 graphene nanoresonator arrays are placed on a 1 μm thick SiN x membrane with 200 nm Au backreflector. The graphene was grounded through Au(100 nm)/Cr(3 nm) electrodes that also served as source-drain contacts. A gate bias was applied through the SiN x membrane between the underlying Si frame and graphene sheet. The temperature-controlled stage contains a feedback controlled, heated silver block that held a 2 mm thick copper sample carrier, with a 100 μm thick sapphire layer used for electrical isolation. The temperature was monitored with a thermocouple in the block, and the stage was held at a vacuum of 1 mtorr. A 1 mm thick potassium bromide (KBr) window was used to pass thermal radiation out of the stage, which was collected with a Cassegrain objective and passed into an FTIR with an MCT detector. ( b ) A representative SEM image of 30 nm graphene nanoresonators on a 1 μm thick SiN x membrane. ( c ) Source-drain resistance versus gate voltage curve of the device. The peak in the resistance occurs at the charge neutral point (CNP), when the Fermi level ( E F ) is aligned with the Dirac point. 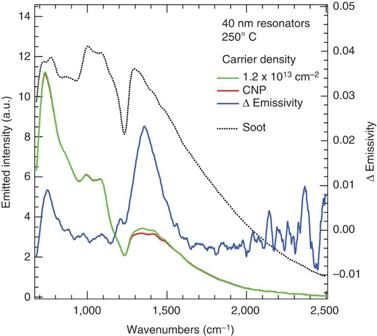Figure 2: Experimental emission results. (Left axis) Emitted thermal radiation at 250 °C from soot (black dotted line) and 40 nm graphene nanoresonators at zero (red) and 1.2 × 1013cm−2(green) carrier density. (right axis, blue line) Change in emissivity of 40 nm nanoresonators due to increase in carrier density. Soot reference is assumed to have emissivity equal to unity. Full size image Tunable emission measurements on graphene nanoresonators Figure 2 (left axis) shows the emitted radiation at 250 °C from a black soot reference sample and from a 40 nm graphene nanoresonator array at 250 °C under doped (1.2 × 10 13 cm −2 ) and undoped conditions. On the right axis of Fig. 2 , we plot the change in emissivity corresponding to the observed change in emitted light from the undoped to doped graphene resonators. This change in emissivity is calculated assuming unity emissivity at all frequencies for the black soot reference and normalizing accordingly. As can be seen in the figure, increasing the carrier density of the graphene nanoresonators leads to increases in emissivity near 730 and 1,400 cm −1 . Figure 2: Experimental emission results. (Left axis) Emitted thermal radiation at 250 °C from soot (black dotted line) and 40 nm graphene nanoresonators at zero (red) and 1.2 × 10 13 cm −2 (green) carrier density. (right axis, blue line) Change in emissivity of 40 nm nanoresonators due to increase in carrier density. Soot reference is assumed to have emissivity equal to unity. Full size image To explore these gate-tunable emissivity features, we investigate their behaviour as the nanoresonator doping and width is varied, as shown in Fig. 3a,b , as well as their polarization dependence ( Fig. 3c ). These results indicate that the intensity, width and energetic position of the thermal radiation feature near 1,360 cm −1 are widely tunable, and that this feature is strongly polarized. The energy of this feature increases as the nanoresonator width is decreased and as the carrier density is increased, while the intensity of this feature increases with carrier density, and is the largest in 40 nm resonators, when it occurs closest to the λ /4 n SiN resonance condition of the SiN x at 1,360 cm −1 . As Kirchoff’s Law dictates that thermal emissivity is equal to absorptivity, these observations are consistent with previously reported absorption measurements performed on identical samples that showed a narrow absorption feature near 1,360 cm −1 [30] (see also Supplementary Note 2 ; Supplementary Fig. 4 ). 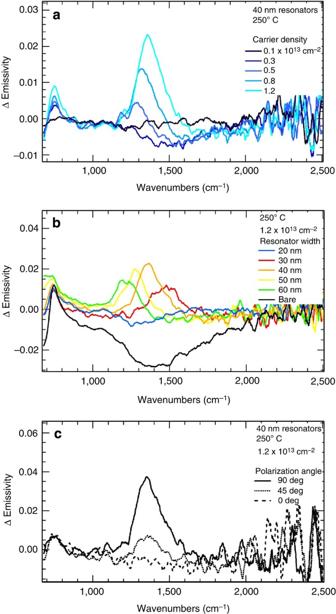Figure 3: Emissivity tunability. (a) Carrier density dependence of change in emissivity with respect to the CNP for 40 nm graphene nanoresonators at 250°C. (b) Width dependence of change in emissivity for 20, 30, 40, 50 and 60 nm wide nanoresonators at 250°C and for a carrier density of 1.2 × 1013cm−2. (black line) Emissivity change for a nearby region of bare, unpatterned graphene at the same carrier density and temperature. (c) Polarization dependence of the emissivity change for 40 nm graphene nanoresonators at 250°C, for a carrier density of 1.2 × 1013cm−2. Figure 3: Emissivity tunability. ( a ) Carrier density dependence of change in emissivity with respect to the CNP for 40 nm graphene nanoresonators at 250°C. ( b ) Width dependence of change in emissivity for 20, 30, 40, 50 and 60 nm wide nanoresonators at 250°C and for a carrier density of 1.2 × 10 13 cm −2 . (black line) Emissivity change for a nearby region of bare, unpatterned graphene at the same carrier density and temperature. ( c ) Polarization dependence of the emissivity change for 40 nm graphene nanoresonators at 250°C, for a carrier density of 1.2 × 10 13 cm −2 . Full size image Low-energy emission feature The lower-energy emissivity modulation feature near 730 cm −1 shows different behaviour than the higher-energy peak. Namely, the low-energy feature shows an extremely weak polarization dependence and also shows no noticeable dependence on graphene nanoresonator width. As the carrier density is increased, there is a small, non-monotonic increase in intensity for this feature, but it shows no spectral shift. Finally, unlike the higher-energy peak, the lower-energy peak is also observed in the bare, unpatterned graphene, where it appears as a slightly narrower feature. The absorption properties of this device near the energy range of the lower-energy feature were not discussed in previously reported work due to the low-energy cutoff of the detector used in that work. We explain the above phenomena as electronic control of thermal radiation due to a combination of plasmon–phonon and plasmon–electron interactions, Pauli-blocking of interband transitions, and non-radiative transfer processes between the SiN x and the graphene sheet. While Kirchoff’s law dictates that the thermal equilibrium emissivity must be equal to the absorptivity for any material, the precise, microscopic mechanisms of thermal emission are markedly modified in inhomogeneous artificial photonic materials with highly confined optical modes relative to homogeneous materials. We attribute the prominent spectral feature at 1,360 cm −1 to a Fabry-Perot plasmonic resonance from the patterned graphene. The width and doping dependence of the 1,360 cm −1 feature follows the behaviour expected for graphene plasmonic modes, and is consistent with reflection measurements [30] . Specifically, the graphene plasmon resonant frequency should vary as ω p ∝ n 1/4 W −1/2 , where n is the carrier density and W refers to the resonator width. This behaviour is in accord with the emission spectra in which we observe a blue shift of the plasmonic resonance at increased doping and decreased graphene nanoresonator width. The intensity of the higher-energy peak increases with graphene carrier density, an effect that results from the increased polarizability of the resonant plasmonic modes. Finally, this feature is strongly polarization dependent, as we would expect for laterally confined graphene plasmonic resonant modes, and vanishes quickly as we rotate the polarization of the probing radiation from 90° to 0° relative to the nanoresonator axis. To understand the source of thermally excited plasmons in graphene nanoresonators, we note that the microscopic processes that lead to plasmonic loss in graphene should by reciprocity correspond to plasmon-generating processes when the sample is heated. For the case of the 1,360 cm −1 feature we observe here, the plasmonic loss (and corresponding plasmon generating) processes are attributed to the factors that limit the electron mobility of the graphene, such as defect scattering, impurity scattering, and inelastic electron–electron and electron–phonon interactions [15] , [22] , [25] , [30] , [33] . In addition, plasmons have been shown to decay via loss channels associated with the edges of graphene nanostructures and by coupling to substrate phonons [22] , [25] . For a bare graphene sheet, the plasmons generated by thermal emission do not couple well to free space and are thus non-radiative. Upon patterning the graphene, however, the plasmonic resonances can effectively serve as antennas that out-couple radiation, and the plasmon decay processes give rise to free-space thermal emission by exciting resonant plasmonic modes that then radiate. The resonant enhancement of emission from plasmon generating processes is in competition with the blocking of interband transitions that act as thermal emitters in the undoped graphene, but are forbidden due to Pauli blocking when the sheet is doped [9] , [10] . The role of interband transitions can be seen most clearly in the bare graphene emissivity spectra in Fig. 3b where there is a broad decrease in emissivity near 1,360 cm −1 at higher carrier densities. While interband transitions should occur across a wide range of frequencies, in the back reflector geometry we use here, thermal emission from the surface can either constructively or destructively interfere with itself and is thus most prominent at 1,360 cm −1 , the λ /4 n SiN frequency of the SiN x layer. For patterned graphene areas, however, we find that doping the graphene allows for the resonant plasmonic modes to create an emission enhancement that outweighs the decrease in emission due to Pauli blocking, and thus we get a net increase in emission near 1,360 cm −1 . As mentioned above, in addition to out-coupling of radiation due to plasmon loss mechanisms in the graphene, the plasmonic resonators also interact with vibrations in the SiN x substrate. When the SiN x is heated, the plasmonic modes act as antennae to enhance the spontaneous thermal radiation from the nearby SiN x . The enhancement of the spontaneous emission radiative rate and of the quantum efficiency arising from dipole emitters’ proximity to a dipole optical antenna is well known [34] , [35] , [36] , and is attributed to increasing the probability of radiative emission by modification of the photonic mode density [37] . The rate enhancement is correlated to the strong polarizability of the graphene at its plasmonic resonance that enhances the outcoupling of thermal radiation from the SiN x . In particular, the radiative rate is expected to be most strongly amplified within the mode volume of the resonant graphene plasmon, which for 40 nm resonators at 1.2 × 10 13 cm −2 roughly corresponds to the area within 10 nm of the resonator (see Fig. 4a ). We therefore assign the net increase of thermal emission near 1,360 cm −1 to a combination of thermal excitations in the graphene as well as thermal phonons in the SiN x that is out-coupled through the confined plasmonic modes in the graphene nanoresonators. 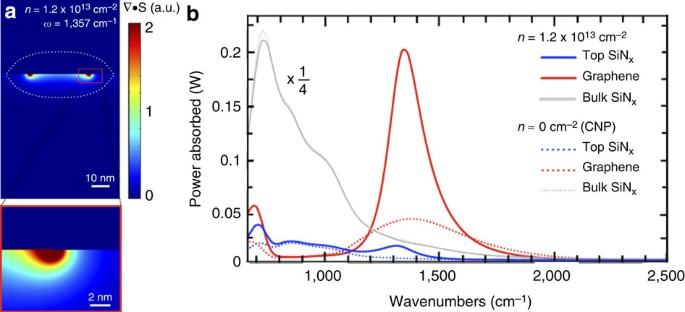Figure 4: Finite element power density simulations. (a) Finite element electromagnetic simulation of(electromagnetic power density) in graphene/SiNxstructure for 40 nm graphene nanoresonators on 1 μm SiNxwith a gold backreflector . The simulation is performed at 1,357 cm−1(on plasmon resonance) at a carrier density of 1.2 × 1013cm−2. Dotted white line indicates the mode volume of the plasmon resonance. (b) Integrated power density absorbed in the 40 nm graphene nanoresonator, the SiNxwithin the plasmon mode volume (Top SiNx), and the remaining bulk of the SiNx(Bulk SiNx) for carrier densities of 1.2 × 1013cm−2and∼0 cm−2(the charge neutral point). Figure 4: Finite element power density simulations. ( a ) Finite element electromagnetic simulation of (electromagnetic power density) in graphene/SiN x structure for 40 nm graphene nanoresonators on 1 μm SiN x with a gold backreflector . The simulation is performed at 1,357 cm −1 (on plasmon resonance) at a carrier density of 1.2 × 10 13 cm −2 . Dotted white line indicates the mode volume of the plasmon resonance. ( b ) Integrated power density absorbed in the 40 nm graphene nanoresonator, the SiN x within the plasmon mode volume (Top SiN x ), and the remaining bulk of the SiN x (Bulk SiN x ) for carrier densities of 1.2 × 10 13 cm −2 and ∼ 0 cm −2 (the charge neutral point). Full size image In contrast to the high-energy feature, which is due to plasmons in the graphene, the low-energy feature at 730 cm −1 is related to an optically active phonon in the SiN x substrate. This phonon mode is strongly absorbing (emitting) and is typically located near 850 cm −1 . The large divergence in the SiN x permittivity due to this phonon, however, creates an additional λ /4 n SiN condition in the structure that leads to a destructive interference effect, resulting in an absorption (emission) maximum at 730 cm −1 . When graphene is placed on top of the SiN x , the intraband and interband transitions in the graphene act to modify the surface impedance of the device. The result is that increasing the doping in the graphene leads to a stronger destructive interference effect, which manifests as larger emission from the SiN x layer (see Fig. 4b ). In addition to direct emission from the SiN x phonon, the graphene plasmons can couple to the SiN x phonons to create new surface phonon plasmon polariton modes [21] , [22] , [25] , [38] . The formation of these modes leads to a modification of the plasmonic dispersion relation, and additional absorption (emission) pathways near and below the energy of the SiN x phonon (see Supplementary Note 3 , Supplementary Fig. 5 ). Emission from the SPPP modes, however, should display some polarization dependence, which was not observed in Fig. 3b ; thus, an increase in direct emission from the SiN x layer likely plays the dominant role in creating the feature at 730 cm −1 . To better understand and quantify the emission features observed in the graphene-SiN x structure, we used a finite element method to calculate the electromagnetic power density associated with plane waves incident on 40 nm graphene nanoresonators on an SiN x /Au substrate. The parameters for our computational model were equivalent to those described in our previous work, where the optical absorption of the device was modelled [30] . As reveals where power is absorbed, it therefore also indicates where far-field thermal emission originates, and an increase in indicates an enhancement of the spontaneous emission intensity of the thermally excited dipoles [30] . The results of these simulations are shown in Fig. 4a at 1,357 cm −1 , corresponding to the resonant energy of the graphene plasmon mode when the carrier density is set to 1.2 × 10 13 cm −2 . It can be seen in this figure that there is a marked increase in the amplitude of near the graphene nanoresonator. On resonance, there is a significant amount of power absorbed directly into the graphene, and it can also be seen that there is a large amount of absorption in the SiN x in the immediate vicinity of the nanoresonator, where the fields of the graphene plasmon mode extend. To further distinguish the relative contributions to thermal emission, we integrate the power densities at 1,357 cm −1 over the graphene, the SiN x within the plasmon mode volume and the remaining SiN x . We calculate the mode volume of our structure as where the numerator is the total stored energy and u 0 is the electromagnetic-energy density at the emitter position, chosen to be sitting directly atop the resonator. We define the boundary of the mode to be centred about the graphene resonator along a contour of constant electric field ( E x ). In Fig. 4b , we show results for undoped and doped nanoresonators. For undoped graphene, we observe weak power absorption in the SiN x near the graphene nanoresonator, and we see only interband transitions contributing to absorption in the graphene itself. As the carrier density is increased to 1.2 × 10 13 cm −2 , absorption in the graphene and the nearby SiN x increases due to excitation of the confined plasmonic mode. The absorption in the bulk of the SiN x layer shows little dependence on graphene carrier density, except at low frequencies, near 730 cm −1 , where absorption decreases with carrier density due to changes in the reflection coefficient at the surface, as described above. We note that our finite element model does not account for the non-radiative processes discussed in other work [39] . Our model indicates how graphene plasmons interact with a homogenous, lossy medium but not the manner in which individual dipoles interact with the graphene sheet, which is another source of non-radiative quenching. To quantify the thermally radiated power of this structure, we consider Planck’s law for spectral radiance using the black soot as a reference with =1, and including our 50 × 50 μm 2 collection area and the 1.51 steradians covered by the 0.65 NA objective. This calculation yields a maximum thermal power modulation of 50 pW cm −1 at 1,360 cm −1 (7.1 μm) for 40 nm resonators at 250 °C doped to a carrier density of 1.2 × 10 13 cm −2 (see Supplementary Fig. 3 ). These calculations indicate that a 1 × 1 mm 2 device could act as an electronically controllable mid-IR source that would modulate 2 μW of power over 100 cm −1 of bandwidth. This compares favourably with commercial mid-IR LEDs at 7 μm, which emit 1.25 μW over similar bandwidths (IoffeLED, OPLED70Sr). The percent change in emitted power at the resonant plasmonic frequency is 7.5%, a value that reflects the large background contribution due to SiN x phonons as well as the low mobility of the graphene sheet, the polarization of the plasmon-assisted radiation and the low dielectric strength of the SiN x at elevated temperatures (see also Supplementary Note 2 ; Supplementary Fig. 4 ). Figure 4 shows that while the SiN x phonons play some role in contributing to the plasmon-assisted radiation, the majority originates in the graphene sheet itself. Thus, by choosing a substrate with a low optical phonon density at the resonant plasmon frequency, such as diamond-like carbon [22] , the background signal could be reduced without significantly suppressing the plasmon-assisted radiation, leading to a larger modulation depth of the emitted power. We also note that the maximum temperature and gate bias applied in these experiments was not limited by the graphene but by the SiN x dielectric, which is known to exhibit Poole-Frenkel tunnelling at high temperatures [32] . By choosing a dielectric that can withstand higher temperatures, such as SiO 2 or diamond-like carbon, devices displaying larger power modulation could be fabricated. Finally, devices fabricated with higher mobility graphene, less edge roughness and with circular resonator geometries (that is, non-polarized) have been predicted theoretically [31] to exhibit tunable absorptivity/emissivity that can vary from 0 to 1 (that is, zero to total absorption) within a narrow frequency range. Such devices would display changes in absorbtivity that equal or exceed those provided by electrochromic devices [40] , while also providing potential for more operation cycles, and higher temperature and higher speeds of operation. In addition to providing utility as a tunable mid-IR source, the physics by which this device operates is distinctly different from conventional laser or LED sources. As thermal radiation is a form of spontaneous emission, the emission rate is increased by the presence of the plasmonic cavity, with the degree of rate enhancement dictated by the ratio between the Q factor and mode volume of the optical cavity (that is, the Purcell factor) [41] . This effect has been explored as a means of increasing LED switching rates by placing the semiconductor emitting layer within either a plasmonic or photonic cavity [42] , [43] , [44] , [45] , [46] . For the case of graphene plasmonic nanoresonators that have highly confined mode volumes, the Purcell factor has been shown to be extremely high, approaching 10 7 , and, thus, the modulation rate of thermal emission from our device could be exceedingly fast, beyond what has been demonstrated with plasmonically enhanced LEDs or lasers [47] . For the device demonstrated here, where the switching and detection speeds are limited by a large electrical RC time constant, and the slow operation speeds of our FTIR-based detector, kHz switching speeds can be demonstrated (see Supplementary Note 4 ; Supplementary Fig. 6 for experimental results). However, careful device design, where the capacitance is minimized and lower resistance contacts are used, could allow for the creation of a mid-IR emitter with ultrafast switching times and a broad range of tunability. Sample fabrication Our measurements were performed on graphene grown on 25 μm thick copper foils using established chemical vapour deposition growth techniques [48] , [49] . The graphene was transferred to a 1 μm thick low-stress SiN x membrane with 200 nm of Au deposited on the opposite side that is used as both a reflector and a backgate electrode. Nanoresonators with widths ranging from 20 to 60 nm were then patterned over 70 × 70 μm 2 areas into the graphene using 100 keV electron beam lithography. Carrier density determination A typical gate-dependent resistance curve for one of our structures is shown in Fig. 1c . The peak in resistance corresponds to the charge neutral point (CNP) of the graphene, where the Fermi level is aligned with the Dirac point and the carrier density is minimized. The carrier density of the resonators was determined by fitting the plasmon peak positions at the highest offset gate voltage (Δ V G = V G − V CNP ) to spectra that were calculated using the finite element method described in the paper and used in previous work [30] . The carrier densities at lower gate voltage offsets were determined using a simple linear capacitor model based on this fitting (that is, n ∼ C × Δ V G ) (See Supplementary Fig. 3 ). Blackbody emission measurements For blackbody emission measurements, the device was connected to a temperature-controlled stage consisting of a 100 μm thick layer of sapphire on 2 mm copper on a heated silver block that can vary in temperature from room temperature to 250 °C. The stage temperature was monitored via a thermocouple mounted in the silver block, and the temperature on the SiN x membrane was confirmed to be no more than 15°C less than the thermocouple temperature by placing a series of temperature indicating laquers (Omegalaq) on an equivalent SiN x membrane. The device and stage were held at a pressure of 1–2 mTorr during emission measurements. Gate-dependent emission spectra were measured using a Fourier transform infrared (FTIR) microscope operating such that emitted light from the heated device passes through a KBr window and is collected in a Cassegrain objective, collimated and passed through the interferometer in the FTIR before being focused on a liquid nitrogen-cooled HgCdTe detector. For polarization-dependent measurements a wire grid polarizer was placed in the collimated beam path. As a reference a SiN x /Au membrane was coated with an optically thick layer of black soot deposited using a candle. Soot is known to be a thermal emitter that approximates an ideal blackbody with emissivity approaching unity across the mid-IR [6] . How to cite this article: Brar, V.W. et al . Electronic modulation of infrared radiation in graphene plasmonic resonators. Nat. Commun. 6:7032 doi: 10.1038/ncomms8032 (2015).